Plant tumour biocontrol agent employs a tRNA-dependent mechanism to inhibit leucyl-tRNA synthetase Leucyl-tRNA synthetases (LeuRSs) have an essential role in translation and are promising targets for antibiotic development. Agrocin 84 is a LeuRS inhibitor produced by the biocontrol agent Agrobacterium radiobacter K84 that targets pathogenic strains of A. tumefaciens , the causative agent of plant tumours. Agrocin 84 acts as a molecular Trojan horse and is processed inside the pathogen into a toxic moiety (TM84). Here we show using crystal structure, thermodynamic and kinetic analyses, that this natural antibiotic employs a unique and previously undescribed mechanism to inhibit LeuRS. TM84 requires tRNA Leu for tight binding to the LeuRS synthetic active site, unlike any previously reported inhibitors. TM84 traps the enzyme–tRNA complex in a novel ‘aminoacylation-like’ conformation, forming novel interactions with the KMSKS loop and the tRNA 3′-end. Our findings reveal an intriguing tRNA-dependent inhibition mechanism that may confer a distinct evolutionary advantage in vivo and inform future rational antibiotic design. Leucyl-tRNA synthetases (LeuRSs) have an essential role in translating the genetic code by ligating leucine (Leu) to the 3′-end of tRNA Leu . The LeuRS aminoacylation reaction is catalysed by a highly conserved catalytic domain encoding a nucleotide-binding Rossman fold, and the class I aminoacyl-tRNA synthetase (aaRS)-defining catalytic peptide sequences, the HIGH and KMSKS motifs [1] , [2] . The reaction is catalysed in a two-step mechanism ( Fig. 1a ): in the tRNA-independent first step, Leu is activated by ATP to form a tightly-bound high-energy intermediate Leu-AMP and release of inorganic pyrophosphate; in the second step, Leu-AMP reacts with the 2′-hydroxyl (-OH) of the terminal ribose at the 3′-end of the tRNA Leu to form Leu-tRNA Leu (ref. 3 ). LeuRSs are also composed of a number of additional domains involved in binding tRNA Leu or in proofreading activities [4] , [5] , [6] , [7] . X-ray crystal structures have been obtained for LeuRSs from both archaeal and bacterial origins in complex with a number of substrates and substrate analogues, including Leu [5] and tRNA Leu (refs 6 , 7 ), a reaction-intermediate analogue of Leu-AMP [5] , and also substrate mimics of both post- and pre-transfer editing reactions [8] . The range of different LeuRS conformations visualized by these studies highlights the complex interplay of these multi-domain enzymes with their substrates. 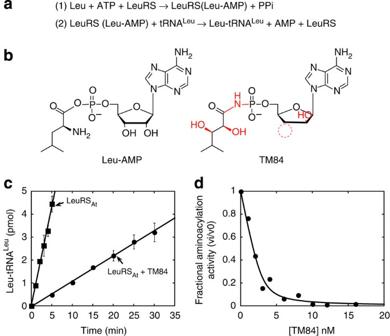Figure 1: TM84 is a tight-binding inhibitor of the LeuRSAtaminoacylation reaction. (a) Aminoacylation reaction of LeuRS. (b) Comparison of Leu-AMP and TM84—differences in red. (c) Inhibition of LeuRSAt(4 nM) aminoacylation reaction +/− TM84 (3 nM). Error bars on the initial rate time points represent standard deviation,n=3. (d) The TM84 dose–response curve of LeuRSAt(4 nM) aminoacylation reaction was fit to the Morrison equation for tight-binding inhibitors (equation (1)), indicating aKi appof 0.3±0.1 nM. Figure 1: TM84 is a tight-binding inhibitor of the LeuRS At aminoacylation reaction. ( a ) Aminoacylation reaction of LeuRS. ( b ) Comparison of Leu-AMP and TM84—differences in red. ( c ) Inhibition of LeuRS At (4 nM) aminoacylation reaction +/− TM84 (3 nM). Error bars on the initial rate time points represent standard deviation, n =3. ( d ) The TM84 dose–response curve of LeuRS At (4 nM) aminoacylation reaction was fit to the Morrison equation for tight-binding inhibitors (equation (1)), indicating a K i app of 0.3±0.1 nM. Full size image LeuRSs, and the other aaRSs, are essential enzymes that are underutilized targets for the development of antibiotics [9] . The most prominent inhibitor class that has been investigated are the rationally designed stable analogues of aminoacyl-adenylates (AA-AMPs) [10] , [11] , [12] , such as leucyl-adenylate sulphamoyl analogue (Leu-AMS), which was used in X-ray crystallographic studies of LeuRS to define the binding pocket of the reaction intermediate [5] . Stable AA-AMP analogues have proven to be potent inhibitors of a range of other aaRSs [13] , [14] . They are thought to act by competing with the amino-acid and ATP substrates for binding to the synthetic active site contained in the catalytic domain, thereby inhibiting the amino-acid activation reaction and consequently aminoacylation. Agrocin 84 is a recently identified inhibitor of LeuRS [15] , [16] . The antibiotic is produced by the biocontrol agent Agrobacterium radiobacter strain K84 that is used worldwide to protect plants against the economically important disease crown gall [17] . The bacterial pathogen A. tumefaciens is the causative agent of the disease and induces tumours into infected plants via the transfer of oncogenic DNA [18] . Agrocin 84 specifically targets strains of A. tumefaciens by acting as a molecular Trojan horse that mimics a plant tumour-derived substrate to gain access into the agrobacterial cell [19] , [20] . Once inside, agrocin 84 is processed into a toxin, TM84, which we have shown to be a potent inhibitor of the A. tumefaciens genome-encoded LeuRS (LeuRS At ) [16] . TM84 closely resembles the obligate reaction intermediate of LeuRSs, Leu-AMP ( Fig. 1b ), but contains a relatively stable N -acyl 5′-phosphoramidate bond instead of the labile phosphoanhydride linkage. We previously hypothesized that TM84 acts as a stable analogue of Leu-AMP and inhibits LeuRS by binding to the synthetic active site [16] . Surprisingly, we now show that TM84 is different from Leu-AMP analogues, as it employs a unique tRNA-dependent inhibition mechanism in which the 3′-end of tRNA Leu is required to form an ‘aminoacylation-like’ conformation that stabilizes the binding of the inhibitor in a ternary inhibition complex. Our structure, together with a recently published structure of an Escherichia coli LeuRS·tRNA Leu ·Leu-AMP analogue [21] , reveal exciting new insights into the recognition of tRNA Leu by LeuRS during aminoacyl transfer, and molecular details of how the enzyme catalyses the second stage of the aminoacylation reaction. TM84 is a tight-binding inhibitor of tRNA Leu aminoacylation To determine the mechanism by which TM84 inhibits LeuRS At , we examined inhibition of the leucylation reaction using an in vitro transcribed substrate encoding the tRNA Leu (UAA) A. tumefaciens isoacceptor. Our results clearly show substantial inhibition of the aminoacylation reaction at concentrations of TM84 ([I]=3 nM) similar to that of the LeuRS At enzyme ([E]=4 nM) ( Fig. 1c ). The stoichiometric levels of TM84 to enzyme required to see inhibition strongly suggested that TM84 is a tight-binding inhibitor of LeuRS At , and therefore required the use of non-Michaelis–Menten kinetic analysis of subsequent inhibition assays to determine the true potency of the inhibitor [22] . Tight-binding inhibitors often display a slow onset of inhibition due to conformational changes of the enzyme on inhibitor binding [23] . This behaviour is typically manifested as a curvilinear appearance to enzyme initial rates that cannot be adequately analysed using the standard discontinuous assays used for aaRSs. To eliminate the potential complexity of slow binding effects on our analysis, TM84 was pre-incubated with the enzyme and tRNA Leu before initiating the aminoacylation reaction. We then plotted the fraction of the aminoacylation rate measured against [TM84] and fit the resulting dose–response curve ( Fig. 1d ) to the Morrison equation for tight-binding inhibitors. The fit showed an apparent K i ( K i app ) of 0.3±0.1 nM, which suggests that TM84 behaves as a tight-binding inhibitor of LeuRS At (ref. 22 ). TM84 weakly inhibits Leu-AMP formation in the absence of tRNA Leu We previously hypothesized that TM84 competes with Leu and ATP for binding to the synthetic active site [16] . To test this, we examined if TM84 could inhibit activation of Leu by ATP in a similar manner to Leu-AMS. We made use of the ATP/pyrophosphate exchange reaction (ATP/PPi), which measures the rate of Leu-AMP formation by the enzyme, in the presence of Leu and ATP substrates, through addition of excess [ 32 P]-labelled inorganic PPi that leads to formation of [γ- 32 P] ATP via a back reaction [24] , [25] . Thus, it is possible to observe the enzyme catalysing multiple turnovers of the Leu activation reaction. As expected, our results show that Leu-AMS is a potent inhibitor of the LeuRS At -catalysed ATP/PPi exchange reaction ( Supplementary Fig. S1 ). Surprisingly, TM84 did not potently inhibit amino-acid activation ( Fig. 2a ). High concentrations of TM84 (limited by availability of this natural product) were required to see even partial inhibition ( Fig. 2b ). 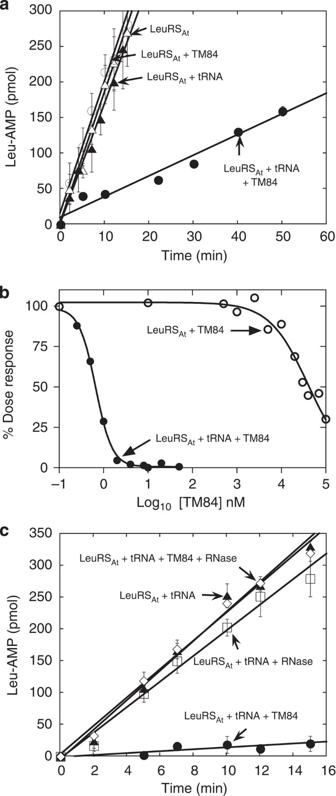Figure 2: tRNALeuis required for reversible TM84 inhibition of leucine activation. (a) TM84 inhibition of LeuRSAt(1 nM) ATP/PPi exchange reaction +/− tRNALeu(6.7 μM). Initial rate reaction conditions are LeuRSAtonly (Δ), LeuRSAtwith 1 μM TM84 (), LeuRSAtwith tRNALeu(▲), and LeuRSAtwith tRNALeuand 50 nM TM84 (). Error bars indicate standard deviation,n=3. (b) TM84 dose–response curves of LeuRSAt-catalysed ATP/PPi-exchange reaction in the absence () and presence () of tRNALeu. IC50 TM84>25 μM and IC50 TM84·tRNA<1 nM. (c) Effect of RNase treatment on LeuRSAt·tRNALeu·TM84 complex ATP/PPi exchange activity. Reaction conditions examined were LeuRSAtwith tRNALeu(▲), LeuRSAtwith tRNALeuand 250 nM TM84 (), preformed LeuRSAt·tRNALeucomplex treated with RNase (), and preformed LeuRSAt·tRNALeu·TM84 complex treated with RNase (). Figure 2: tRNA Leu is required for reversible TM84 inhibition of leucine activation. ( a ) TM84 inhibition of LeuRS At (1 nM) ATP/PPi exchange reaction +/− tRNA Leu (6.7 μM). Initial rate reaction conditions are LeuRS At only (Δ), LeuRS At with 1 μM TM84 ( ), LeuRS At with tRNA Leu (▲), and LeuRS At with tRNA Leu and 50 nM TM84 ( ). Error bars indicate standard deviation, n =3. ( b ) TM84 dose–response curves of LeuRS At -catalysed ATP/PPi-exchange reaction in the absence ( ) and presence ( ) of tRNA Leu . IC 50 TM84 >25 μM and IC 50 TM84·tRNA <1 nM. ( c ) Effect of RNase treatment on LeuRS At ·tRNA Leu ·TM84 complex ATP/PPi exchange activity. Reaction conditions examined were LeuRS At with tRNA Leu (▲), LeuRS At with tRNA Leu and 250 nM TM84 ( ), preformed LeuRS At ·tRNA Leu complex treated with RNase ( ), and preformed LeuRS At ·tRNA Leu ·TM84 complex treated with RNase ( ). Full size image A potential explanation of how TM84 can be a strong inhibitor of the overall aminoacylation, yet not the Leu activation reaction, could be a requirement for tRNA Leu in the inhibition mechanism. To test this, we examined if TM84 inhibition of the LeuRS At aminoacylation activity could be reduced using low concentrations of tRNA Leu substrate. However, the low concentrations of tRNA required to see activity in these assays made quantitation of Leu-tRNA Leu difficult, even when sensitive TLC-based assays were used. To circumvent this, we explored the requirement for tRNA Leu in the inhibition mechanism of TM84 by adding in vitro transcribed tRNA Leu to the ATP/PPi-exchange reaction. This approach has been used before for aaRS enzymes such as glutaminyl- [26] and glutamyl-tRNA synthetases [27] , which, unlike LeuRSs, require tRNA for the activation reaction to proceed. Importantly, in these experiments we used an active tRNA Leu concentration of 6.7 μM that had no effect on the initial rate of ATP/PPi exchange for the LeuRS At reaction ( Fig. 2a ). In addition, negligible amounts of Leu-tRNA Leu , the product of the aminoacylation reaction, were detectable under these reaction conditions ([LeuRS At ]=1 nM ( Supplementary Fig. S2 )). Our experiments were performed +/− tRNA Leu and by varying the [TM84]. The resulting dose–response data were analysed as detailed previously [28] and showed a greater than 4 orders of magnitude increase in the inhibition of the amino-acid activation reaction with tRNA Leu compared to that without tRNA Leu (IC 50 TM84 =>25 μM and IC 50 TM84·tRNA =0.7±0.1 nM; see Fig. 2b ). These results were strongly suggestive that tRNA Leu actively participates in the inhibition mechanism of TM84 for LeuRS At , but also did not rule out that TM84 binds to an alternative site on the enzyme. Some tight-binding enzyme inhibitors form covalent bonds with protein residues (or RNA substrates), leading to irreversible interactions [22] , [29] . To determine if this was the case with the interaction of TM84 with LeuRS At , we pre-incubated LeuRS At with TM84 and tRNA Leu and then added an RNase cocktail to degrade the tRNA into mononucleotides. We then tested samples that had both been incubated +/− RNase for activity in the ATP/PPi exchange experiment. The presence of tRNA potently inhibited the LeuRS At Leu activation reaction, whereas RNAse treatment completely restored activity in the presence of TM84 ( Fig. 2c ). This experiment demonstrates that TM84 binds reversibly to LeuRS At and also supports the idea that tRNA is essential for the tight binding of TM84 to LeuRS At . tRNA Leu increases the binding affinity of TM84 for LeuRS At To gain further insights into the unusual ternary inhibitor interaction, we employed isothermal calorimetry (ITC) to test the effect of tRNA Leu on the energetics of TM84 binding to LeuRS At . Initially, we examined the two separate binding reactions of TM84 ( Fig. 3a ) and tRNA Leu to LeuRS At ( Table 1 ). The two isotherms obtained for binding of TM84 to LeuRS At and tRNA Leu to LeuRS At both fit to single-site binding models with stoichiometries close to 1, and with a calculated K d TM84 of 152±20 nM and a K d tRNA of 84.9±6.1 nM. We then examined the ternary equilibria after pre-incubation with tRNA Leu ( Fig. 3a ). For these experiments, tRNA was first pre-bound to the protein in the ratio of 1.2:1. TM84 was then titrated into the protein–tRNA mixture to obtain the LeuRS·tRNA Leu ·TM84 complex. Surprisingly, the isotherms of the ternary equilibrium exhibited distinct biphasic forms that could not be fitted to a simple single-site model. Instead, the data could be successfully fitted to an independent two-site model with two TM84 binding sites with two different affinities of 0.81±0.31 nM ( K d1 ) and 14.4±1.37 nM ( K d2 ). Although a possible explanation for these results might be that the presence of tRNA creates a second TM84 binding site on the LeuRS At ·tRNA complex, this is not possible as the total stoichiometry of binding in this case would be close to 2. Our data reveal stoichiometric values for the two binding events, n 1 and n 2, summing close to 1 ( n 1+ n 2≈1). Biphasic isotherms can be observed in heterotropic ligand-binding interactions to proteins that display co-operative ligand binding if one of the ligands is present at subsaturating concentration [30] . However, this possibility can be ruled out as the tRNA concentration is saturating. Our results therefore suggest that, rather than observing two independent sites for TM84 on one protein, we are seeing the binding of TM84 to two distinct populations of LeuRS At ·tRNA Leu with two different affinities for TM84. 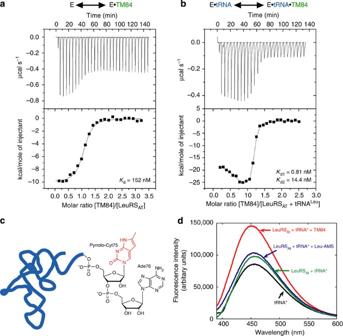Figure 3: tRNA induces TM84 tight-binding and adopts the modified conformation. (a) ITC titration of TM84 into LeuRSAt. The top panel shows raw thermogram and bottom panel shows the binding isotherm fitted to a single-site model (seeTable 1for thermodynamic values). (b) Titration of TM84 into LeuRSAt·tRNALeucomplex. Bottom panel isotherm fitted to a two-independent-sites model. (c) Fluorescent tRNApyrLeuprobe sensitive to the environment of the CCA 3′-end. Pyrrolo-Cyt base (red) located at nucleotide Cyt75. (d) Fluorescence emission spectra for tRNApyrLeu(tRNA*) free or bound to different LeuRSAtcomplexes. Figure 3: tRNA induces TM84 tight-binding and adopts the modified conformation. ( a ) ITC titration of TM84 into LeuRS At . The top panel shows raw thermogram and bottom panel shows the binding isotherm fitted to a single-site model (see Table 1 for thermodynamic values). ( b ) Titration of TM84 into LeuRS At ·tRNA Leu complex. Bottom panel isotherm fitted to a two-independent-sites model. ( c ) Fluorescent tRNApyr Leu probe sensitive to the environment of the CCA 3′-end. Pyrrolo-Cyt base (red) located at nucleotide Cyt75. ( d ) Fluorescence emission spectra for tRNApyr Leu (tRNA*) free or bound to different LeuRS At complexes. Full size image Table 1 Isothermal titration calorimetry data showing binding of TM84 and/or tRNA Leu to LeuRS At . Full size table A mixed population of LeuRS At ·tRNA Leu complexes could originate in two ways. First, single-nucleotide resolution PAGE analysis of the transcript shows ~11% of tRNAs with an additional nucleotide ( N +1) added to the 3′-ends. This is a known side reaction of T7 RNA polymerase when catalysing in vitro transcription reactions [31] . Second, partially misfolded species, perhaps owing to lack of tRNA modifications, are also known to lead to lower percentages of tRNA transcripts that can be aminoacylated. In our case, only ~50% of the tRNA Leu transcripts could be aminoacylated. Interestingly, binding of tRNA Leu to LeuRS At produces a monophasic isotherm, suggesting that the different tRNA Leu species have similar affinities for the enzyme that are indistinguishable from each other in the isotherm. However, the subsequent binding of TM84 can discriminate between the different LeuRS At ·tRNA Leu complexes, giving rise to biphasic isotherms reflecting different binding events. A comparison of the isotherms indicates that TM84 is a relatively weak binder ( K d =152±20 nM) to LeuRS At alone compared to binding to the enzyme pre-incubated with tRNA Leu ( K d =0.81±0.31 nM high-affinity complex). The analysis indicates that binding of TM84 is enhanced up to ~200-fold in the presence of tRNA. If two different LeuRS At ·tRNA Leu complexes are considered, heterotropic interaction constants of 190 and 11 for each complex can be estimated from the ITC experiments [30] , which correspond to cooperativity Gibbs energies of −3.1 and −1.4 kcal mol −1 , respectively. Therefore, tRNA Leu binding to LeuRS adds a 30% increase to the binding Gibbs energy for TM84. These findings are consistent with the results from our kinetics experiments that implicate tRNA Leu in the inhibition mechanism of TM84. TM84 binding to LeuRS·tRNA alters CCA 3′-end conformation The ITC results suggest that catalytically active tRNA and its CCA 3′-end may have an important role in facilitating the tight binding of TM84 in the ternary inhibition complex. To test this, we constructed a tRNA incorporating a fluorescent probe that is sensitive to the conformation and environment of the 3′-terminal nucleotides. We exchanged the penultimate Cyt75 residue of tRNA Leu with a fluorescent pyrrolo-cytidine nucleotide ( Fig. 3c ). This approach was used to monitor the conformation of the CCA 3′-end of tRNA Cys interacting with cysteinyl-tRNA synthetase [32] . By monitoring the fluorescence from this probe, we expected to see a significant change in the spectrum when the LeuRS·tRNApyr Leu complex was bound to TM84 or not. E. coli CCA nucleotidyl transferase was used to catalyse the addition of ATP and pyrCTP onto a truncated in vitro transcribed tRNA Leu (UAA) sequence from A. tumefaciens . Importantly, the fluorescently labelled tRNApyr Leu was a substrate (if somewhat reduced in activity) for the aminoacylation reaction of LeuRS At , indicating that the probe did not disrupt the interaction of the CCA 3′-end with the enzyme. We examined the fluorescence spectra of tRNApyr Leu alone, and in the presence of LeuRS At +/−TM84 or Leu-AMS. The emission fluorescence spectrum of tRNA Leu bound to LeuRS At shows a λ max of 456 nm ( Fig. 3d ). Addition of Leu-AMS to the protein–tRNA complex produces a fluorescence spectrum with similar intensity. However, addition of TM84 both increases the fluorescence intensity (~1.5-fold) and shifts the λ max by 5 nm. This unique TM84-induced spectral signal suggests that the toxin causes a rearrangement of the CCA 3′-end of the tRNA when bound to the LeuRS enzyme. Interestingly, this conformation of the CCA 3′-end of the tRNA does not appear to be substantially populated in the LeuRS·tRNApyr Leu ·Leu-AMS ternary complex. Structure of the LeuRS·tRNA Leu ·TM84 inhibition complex To understand how TM84 binds to LeuRS and gain structural insights into the role of tRNA Leu in the unusual LeuRS inhibitory properties of TM84, we crystallized LeuRS in complex with tRNA Leu and TM84. We used recombinant E. coli LeuRS (LeuRS Ec ) and in vitro transcribed E. coli tRNA Leu (UAA) isoacceptor substrates, which have recently been shown to produce high diffraction-quality crystals [21] . Importantly, LeuRS Ec shares 46% sequence identity with, and has similar domain architecture to, LeuRS At ( Fig. 4a ). LeuRS Ec has similar steady-state kinetic properties to that of LeuRS At ( Supplementary Table S1 ) and aminoacylation by LeuRS Ec is potently inhibited by TM84 ( Supplementary Fig. S3 ). The crystal structure of the LeuRS Ec ·tRNA Leu ·TM84 complex was solved by molecular replacement using the core of the complex formed by Thermus thermophilus LeuRS (LeuRS Tt ) with tRNA Leu [6] , followed by building of the insertion domains. The model was refined to a final R -factor of 18.2% ( R -free=23.6%) at a final resolution of 2.4 Å ( Fig. 4b ; Table 2 ). The asymmetric unit contained two molecules of the ternary complex LeuRS·tRNA Leu ·TM84, one with slightly higher B -factors than the other. 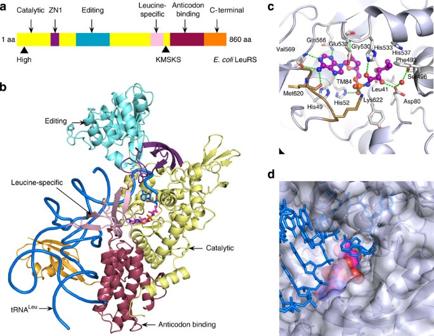Figure 4: Structure of the LeuRSEc·tRNALeu·TM84 inhibition complex. (a) Domain structure of LeuRSEc. (b) Structure of LeuRSEc·tRNALeu·TM84 complex in ‘aminoacylation-like’ conformation. Domains coloured and labelled, tRNALeu(blue) with Ade76 and TM84 depicted with stick bonds in synthetic active site. (c) Active site interactions with TM84. (d) Encapsulation of TM84 (space filling model—pink) in synthetic active site. LeuRSEcprotein surface—grey and tRNALeu—blue. Figure 4: Structure of the LeuRS Ec ·tRNA Leu ·TM84 inhibition complex. ( a ) Domain structure of LeuRS Ec . ( b ) Structure of LeuRS Ec ·tRNA Leu ·TM84 complex in ‘aminoacylation-like’ conformation. Domains coloured and labelled, tRNA Leu (blue) with Ade76 and TM84 depicted with stick bonds in synthetic active site. ( c ) Active site interactions with TM84. ( d ) Encapsulation of TM84 (space filling model—pink) in synthetic active site. LeuRS Ec protein surface—grey and tRNA Leu —blue. Full size image Table 2 Data collection and refinement statistics. Full size table The overall structure of the LeuRS Ec ·tRNA Leu ·TM84 complex ( Fig. 4b ) is very different from the previously described editing conformation of bacterial LeuRS [6] . Remarkably, it shows that the tRNA Leu acceptor stem is present in an ‘aminoacylation-like’ conformation, with the CCA 3′-end penetrating into the synthetic active site of LeuRS Ec where TM84 is bound ( Fig. 4b ; Supplementary Figs. S4, S5a ). This suggests that TM84 causes inhibition of LeuRSs by resembling a stable form of Leu-AMP and thus prevents binding of the Leu and ATP substrates [16] . This finding also weakens an alternative hypothesis that proposes that the unusual inhibitory properties of TM84 are caused by the inhibitor binding to an alternative site on the enzyme other than the synthetic active site [8] , [33] . The most striking feature of the TM84 ternary structure is the pronounced movement of the highly conserved KMSKS loop across the active site of the enzyme when compared with previous LeuRS Tt structures bound to adenylate analogues [5] , [8] or tRNA [6] ( Fig. 4d ). The synthetic active site where TM84 is located is almost completely covered, encapsulating the ligand and presumably decreasing the dissociation rate of the inhibitor from the enzyme. The closed conformation of the KMSKS loop allows new protein–tRNA interactions that stabilize the aminoacylation conformation of the tRNA, notably the hydrogen bonds between the side chain of Lys619 and both the base of Cyt75 and phosphate of Gua71 ( Supplementary Fig. S5a,b ). Indeed, the structure shows that substantial re-ordering of the active site is mandatory for TM84 to form its ‘aminoacylation-like’ ternary complex. Interestingly, this is a property found in slow, tight-binding enzyme inhibitors [23] . To identify key interactions in the LeuRS ternary complex that may be responsible for the tRNA-dependence of TM84 binding, we made comparisons with a structure of LeuRS Ec ·tRNA Leu ·Leu-AMS captured in the functional aminoacylation conformation [21] . Leu-AMS, unlike TM84, does not show tRNA-dependent binding to LeuRS and as a consequence the tRNA could occupy more than one conformation on the enzyme in solution, an observation that is in accordance with our fluorescence data ( Fig. 3d ). Interestingly, the average B factors obtained from both structures do not reveal significant differences in the overall mobility of the two proteins in the crystal nor when individual B factors for domains are compared. A close comparison between the binding mode of TM84 ( Fig. 4c ) and Leu-AMS in their respective LeuRS Ec ·tRNA Leu ‘aminoacylation-like’ ternary complexes identifies a number of shared interactions between both ligands (His52, Phe493, Gly530, Glu532, His533, His537, Gln566, Val569 and Met620), but also reveals key variations between the binding mode exhibited by the two ligands ( Fig. 5a–c ) that could explain their fundamental difference in tRNA-dependency. The chemical structures of TM84 and Leu-AMS are different, which is reflected in the differential binding and inhibition behaviours exhibited by the two molecules. In TM84, the Leu side-chain is replaced by a substituted methyl pentanamide with an OH group (C2-OH) replacing the α-amino group and an additional OH group on the side-chain (C3-OH) ( Fig. 1b ). The C2-OH of the methyl pentanamide group of TM84 forms a hydrogen bond with Asp80, mimicking the interaction with the α-amino group as in the Leu-AMS bound protein. However, the main chain carbonyl oxygen of Leu41 hydrogen bonds to the C3-OH of TM84 ( Fig. 5a ), whereas in the Leu-AMS complex, it only hydrogen bonds with the α-amino group ( Fig. 5b ). TM84 also contains a 3-deoxyarabinose sugar ring substituting for the ribose found in Leu-AMP/Leu-AMS. In the Leu-AMS-bound structure, the ribose 2′-OH and 3′-OH groups, each make a hydrogen bond with active site residue Gly530 ( Fig. 5b ). However, the loss of the cis -diol from the TM84 sugar results in only a single hydrogen bond between its 2′-OH group and Gly530 that extends above the plane of the sugar ring ( Fig. 5a ). Perhaps the most striking and intriguing difference between the two ternary complexes is in the ribose pucker of the terminal adenosine (Ade76). In the Leu-AMS functional aminoacylation state, this ribose is in a C2′- exo conformation, allowing the 2′-OH to point towards the carbonyl-carbon of Leu-AMS ( Fig. 5b ) as would be expected prior to the transfer step in the aminoacylation reaction [21] . In the TM84 complex, the Ade76 ribose is in an unexpected C2′- endo conformation, resulting in the 2′-OH pointing away from the carbonyl-carbon and instead forming a hydrogen bond to a nearby water molecule that in turn hydrogen bonds to Asp80 and Ser496 ( Fig. 5a ). The altered position of the 3′-OH allows it to make a direct hydrogen bond to the C2-OH of TM84. This direct interaction between tRNA Leu and TM84 may play an additional role in stabilizing the ternary inhibition complex. 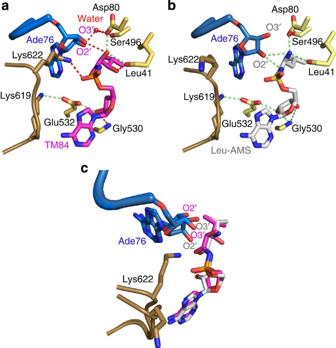Figure 5: Comparison of TM84 and Leu-AMS bound in LeuRSEcternary complexes. (a) TM84 (pink) binding in the synthetic active site showing interactions with the KMSKS loop (gold) and the terminal tRNA Ade76 (blue). The ribose of the adenosine is in the C2′-endoconformation. Water molecule depicted as a red sphere. (b) Leu-AMS (grey) in its respective ternary complex. The ribose of the adenosine in this structure is in the C2′-exoconformation. (c) Superimposition of the two ligands in their respective ternary complexes. Figure 5: Comparison of TM84 and Leu-AMS bound in LeuRS Ec ternary complexes. ( a ) TM84 (pink) binding in the synthetic active site showing interactions with the KMSKS loop (gold) and the terminal tRNA Ade76 (blue). The ribose of the adenosine is in the C2′- endo conformation. Water molecule depicted as a red sphere. ( b ) Leu-AMS (grey) in its respective ternary complex. The ribose of the adenosine in this structure is in the C2′- exo conformation. ( c ) Superimposition of the two ligands in their respective ternary complexes. Full size image Importantly, there is also a significant difference between the KMSKS loop conformation for the two ligands. Whereas in the Leu-AMS ternary complex the second Lys of the K 619 MSK 622 S loop (Lys622) points away from the active site ( Fig. 5b ), in the TM84 complex Lys622 points right into the active site and interacts with a non-bridging oxygen of the negatively charged N -acyl phosphate group of TM84 ( Fig. 5a ; Supplementary Fig. S5b ). The positioning of Lys622 is also a contributing factor in the reduced solvent accessibility of TM84 when bound to the LeuRS Ec (20.6 Å 2 ) compared to Leu-AMS (44.2 Å 2 ). Several factors may contribute to the different conformations exhibited by Lys622 in the two structures. First, the insertion of positively charged Lys622 into the active site is electrostatically favoured both by the presence of the charged N -acyl phosphate group and by the absence of the α-amino group in the case of TM84. In contrast, for Leu-AMS, the sulphate is uncharged. Second, the particular C2′- endo ribose pucker of Ade76 in the TM84 complex avoids potential steric hindrance of Lys622 entering the site, which would be the case with the functional C2′- exo conformation. Interestingly, His52, the second histidine residue of the H 49 IGH 52 catalytic motif, makes an interaction with the other non-bridging oxygen of the phosphate moiety of TM84 ( Fig. 4c ). Although the ionic interaction between Lys622 and the α-phosphate of TM84 is not seen in other LeuRS structures bound to the adenylate analogue (but it remains to be seen what would happen with the true negatively charged Leu-AMP), an equivalent interaction was found in a GlnRS·tRNA Gln ·Gln-AMS ‘aminoacylation’ structure [10] . However, the conformation of the KMSKS loop in this structure does not close so fully over the synthetic active site as in the LeuRS ternary complexes. The observed position of the second lysine of the KMSKS catalytic peptide in the TM84 complex more resembles the conformation expected for the amino-acid activation reaction, as this residue is known to have an important role in both catalysis of activation and the binding of the α and γ phosphates of ATP [34] . Our biophysical and biochemical analyses elucidate a new tRNA-dependent LeuRS inhibition mechanism for TM84, which clearly distinguishes it from Leu-AMS. The crystal structure of the TM84 ternary complex, however, only reveals subtle differences. The binding of TM84 to the LeuRS At active site in the absence of tRNA is considerably weaker than that observed for Leu-AMS. A number of interactions found in Leu-AMS-bound structures [5] , [21] that are absent when TM84 is bound ( Figs. 4c , 5a ) may explain the reduced affinity of TM84 for LeuRS At in the absence of tRNA. These include loss of hydrogen bonds to the sugar moiety of the nucleotide and loss of a potential ionic interaction with Leu-AMS when its amino group is replaced with a hydroxyl in TM84. The crystal structure also reveals three additional interactions that are formed in the presence of tRNA: Lys619 to Cyt75; Lys622 to the phosphate of TM84; and Ade76 to TM84 ( Supplementary Fig. S5b ). We hypothesize that absence of tRNA and concomitant loss of two of these interactions lead to increased KMSKS loop mobility, and destabilization of the Lys622 interaction with TM84. The role of tRNA and the KMSKS loop in binding TM84 also raises kinetic questions about the exact order of binding events. TM84 has to bind to an open active site prior to the positioning of the CCA 3′-end in the final closed ternary complex, leading to decreased dissociation of TM84 (slow k off rate). What is not clear, is how rapidly TM84 binds to the open active site ( k on ); how tRNA might affect this initial binding event; or whether the KMSKS loop binds to TM84 independently of the CCA 3′-end or not. Pre-steady-state kinetic analysis is required to determine the precise order of these events. Why would nature evolve a Trojan Horse LeuRS inhibitor [16] with a tRNA-dependent inhibition mechanism? Perhaps when LeuRS At is inhibited, substrate concentrations would be expected to rise in agrobacterial cells. Under these conditions, a simple LeuRS competitive inhibitor might have decreased toxicity, whereas the higher concentrations of deacylated tRNA Leu would increase the affinity of TM84 for the enzyme. Whatever the reason, this study provides insight into a novel tRNA-dependent inhibitor of LeuRS with potential ramifications for rational antibiotic design. Protein expression and purification LeuRS At was expressed in E. coli BL21 (DE3) RIL codon plus cells containing the pET-21b plasmid encoding LeuRS At with a carboxy-terminal 6X-histidine tag (the leuS At gene had been subcloned in to pET-21b using Nde I and Xho I restriction sites) [16] . Cells were grown in Luria broth at 37 °C, with appropriate antibiotics, to an optical density of 0.3–0.4 (measured at A 600 ) before induction with 1 mM isopropyl-B- D -thiogalactopyranoside. The cells were grown for an additional 3–4 h at 24 °C before harvesting by centrifugation at 5,400 g for 10 min. Cells were lysed by sonication in standard Qiagen lysis buffer. The soluble His-tagged LeuRS At protein was purified using Ni-NTA agarose (Qiagen) as detailed by the manufacturer. The protein was further purified by FPLC using a Mono-Q column and a gradient of 20 mM NaCl to 500 mM NaCl in Tris–HCl buffer (pH 8.0). The purified protein was confirmed to be >95% pure using SDS–polyacrylamide gel electrophoresis. Active LeuRS At protein concentration for kinetic assays was determined by active site titration (see below). LeuRS Ec used for structural studies was expressed in E. coli BL21 cells containing pET-15b plasmid encoding LeuRS Ec with an amino-terminal 6X-histidine tag (MGSSHHHHHHSSGLVPRGSH) under similar conditions [21] . TM84 purification Agrocin 84 (purified as detailed previously [16] ) was incubated in sodium phosphate buffer (pH 7.0) at 100 °C for 15 min and the liberated TM84 toxin was separated from other reaction products by reverse-phase high-performance liquid chromatography. The concentration of purified TM84 was determined using an extinction coefficient ( ε 260 nm ) of 0.0154 M −1 cm −1 . tRNA Leu transcription Plasmids encoding tRNA Leu (UAA) isoacceptor sequences from A. tumefaciens C58 or E. coli in front of T7 polymerase promoter sequences were purified from E. coli DH5-α cells before digestion overnight at 60 °C with Bst NI restriction enzyme to linearize the plasmid DNA. The transcription reaction was performed using template DNA (450 μg), 9 μM T7 RNA polymerase [35] , 1 U ml −1 RNAse inhibitor, 40 mM Tris-HCl (pH 8.0), 25 mM MgCl 2 , 40 mM DTT, 0.1% Triton X-100, 1 mM spermidine and 2 mM rNTPs. The reaction mix was incubated at 37 °C overnight before quenching with 50 mM EDTA followed by DNase I digestion for 1 h to remove template DNA. Phenol–chloroform extraction (pH 5.2) followed by ethanol precipitation (using 0.3 M sodium acetate) isolated the tRNA from the reaction. The precipitated tRNA was gel purified on a 12% denaturing polyacrylamide gel electrophoresis (19:1), 8 M urea gel and 1 × Tris–borate EDTA buffer (pH 8.3). After gel extraction, elution and ethanol precipitation, the purified tRNA Leu (UAA) was refolded by denaturing at 95 °C for 1 min, followed by addition of 1 mM MgCl 2 , and gradually cooled to 28 °C for 1 h. The concentration of refolded tRNA Leu was determined using a theoretical extinction coefficient ( ε 260 ) of 531,500 M −1 cm −1 modified by a factor of 1.34 to account for the hypochromic effect of tRNA folding on absorbance. Active site titration assay The concentration of active LeuRS enzyme for kinetic assays was determined by active site titration as described previously [25] . The reaction buffer contained 50 mM HEPES buffer (pH 7.4), 20 mM KCl, 10 mM MgCl 2 , 10 mM β-mercaptoethanol (β-ME), 1 mM L-Leu, 5 μg/ml inorganic pyrophophatase, 5 μM ATP, 4 μCi [γ- 32 P] ATP and purified recombinant LeuRS enzymes ranging in total protein concentration from 1 to 2 μM (determined by Biorad Protein assay). The reaction was carried out at 28 °C and 5 μl time point aliquots collected. The assay was performed in triplicate and the active enzyme concentration was determined by measuring the amplitude of the burst phase of Leu-AMP formation [24] , [25] . ATP/PPi exchange assay The ATP/PPi exchange assays were performed as detailed earlier [25] . Reaction mixtures containing 50 mM HEPES buffer (pH 7.4), 20 mM KCl, 10 mM MgCl 2 , 500 μM L-Leu, 4 mM ATP, 1 mM tetrasodium pyrophosphate (NaPPi), 10 μCi mmol −1 [ 32 P] NaPPi, 1 μM bovine serum albumin and LeuRS At (1–2 nM) were incubated at 28 °C. LeuRS At enzyme was pre-incubated for 1 h with inhibitor +/− tRNA Leu (6.7 μM) in appropriate experiments and the reactions were initiated by addition of 4 mM ATP and incubated at 28 °C (LeuRS At ) or 37 °C (LeuRS Ec ). Five-microlitre aliquots for each time point were collected, acid quenched and processed [25] . The amount of [ 32 P]-PPi incorporation into ATP was measured by liquid scintillation counting. Aminoacylation assay The 40-μl leucylation reaction mixtures contained 50 mM HEPES (pH 7.4), 20 mM KCl, 25 mM MgCl 2 , 25 mM β-ME, 4 mM ATP, 500 μM [3,4,5- 3 H] L-Leu (20 μCi mmol −1 ), 5 μg/ml inorganic pyrophosphatase and 13.4 μM of active in vitro transcribed tRNA Leu (50% tRNA Leu (UAA) is active based on tRNA charging at saturating enzyme and substrate concentrations). Reactions were initiated with 1–8 nM of active LeuRS enzyme that had been pre-incubated for 1 h with the tRNA Leu substrate +/− inhibitor. Reactions were incubated at 28 °C (LeuRS At ) or 37 °C (LeuRS Ec ). Five-microlitre aliquots of the reaction mix were spotted on 5% trichloroacetic acid (TCA) pre-soaked filter pads, washed twice with 5% TCA and then with 70% ethanol at 4 °C. The pads were dried and quantified using scintillation counting. Initial rates (within the first 10–15% part of the reaction) were obtained and an average rate from three individual data sets was used to plot the dose–response curve, which was fit to a standard form of the Morrison equation for tight-binding inhibitors (see below). Morrison equation: Steady-state fluorescence The penultimate base of the appropriate tRNA Leu (UAA) isoacceptor was labelled with a pyrrolo-cytidine fluorophore. To achieve labelling, E. coli tRNA nucleotidyl transferase enzyme was incubated with a truncated in vitro tRNA transcript and pyrrolo-CTP (Trilink Biotechnologies) and ATP as outlined previously [32] . Fluorescence experiments were performed in buffer containing 50 mM HEPES (pH 7.4), 20 mM KCl, 10 mM MgCl 2 and 10 mM β-ME at 28 °C. Briefly, 0.2 μM pyrrolo-C labelled fluorescent tRNA Leu (UAA) isoacceptor was added to 1 μM LeuRS At , and 2.5 μM TM84 or Leu-AMS. The fluorescence spectra were collected on a Horiba Fluoromax-2 fluorimeter. The excitation wavelength was 352 nm and emission was measured between 390–600 nm. Excitation and emission slit widths were both 5 nm. The spectra were analysed with Datamax software and corrected with appropriate blanks to obtain the final spectra. Isothermal titration calorimetry TM84 interactions with LeuRS At were explored using a VP-ITC and an Auto-ITC200 microcalorimeter (MicroCal/GE Healthcare). All solutions were prepared in buffer containing 50 mM HEPES (pH 7.4), 20 mM KCl, 10 mM MgCl 2 and 1 mM β-ME. For thermodynamic experiments, LeuRS At active protein concentration was determined using ITC titration of a tight-binding ligand (Leu-AMS) to LeuRS At as detailed elsewhere [36] . LeuRS At (active protein concentrations ranging from 4 to 8 μM) was placed in the sample cell and the ligand (at a concentration 10-fold higher than that of the protein) was placed in the syringe. In the ternary titrations, tRNA Leu was added to LeuRS in the cell at a 1:1.2 molar ratio. Titrations were carried out at pH 7.4 and 28 °C. The injection volume was 5–15 μl and the time between injections was 180–240 s. The data were analysed using Origin for ITC software (version 7), and fitted to a one-site or a two-site binding model (due to mixing artefacts, the heat associated with the first peak was excluded from the data analysis). Binding affinity ( K d ), stoichiometry ( N ) and enthalpy (Δ H ) for each complex were determined. The c -values (=[ P total ] × K a ) in our experiments varied from 4 to 900, well within the suggested range of 1–1,000 (ref. 37 ). Crystallization and X-ray data collection To crystallize the LeuRS Ec ·tRNA Leu ·TM84 complex, a 2-μl aliquot of the solution containing the complex was mixed with 2 μl of a crystallization solution and then equilibrated by hanging-drop vapour diffusion against 500 μl of reservoir solution. Crystals appeared at 273 K within 4–5 days in 0.1 M Bis-TRIS at pH 5.5 and 23–25% PEG 3350. For data collection, crystals were flash-cooled directly in liquid nitrogen. Diffraction data were collected at 100 K at the European Synchrotron Radiation Facility on beamline ID14-EH4 (ESRF, Grenoble, France). Crystals were of space-group C 2 with two molecules of complex per asymmetric unit. Data sets were integrated and scaled using the XDS suite [38] . Subsequent data analysis was performed with the CCP4 suite. Structure determination and refinement The structure was solved by molecular replacement (PHASER [39] ) using the core of the protein from the LeuRS Ec editing complex (1–223, 416–568 and 795–860 residues [21] . The resulting model was used to search for the core of the tRNA (bases 5–79) and to manually build the external flexible domains using COOT [40] . The Zn domain (158–189), not visible in the LeuRS Ec editing complex, was built using the analogous T. thermophilus LeuRS structure as a guide. Models were refined by rigid-body refinement, followed by isotropic B -factor refinement using REFMAC5 with translation libration screw-motion [41] . In the resultant 2 m | F o |− D | F c | and m | F o |− D | F c | maps, we clearly found both tRNA and TM84 electron densities. The crystallographic data collection and final refinement statistics are presented in Table 1 . Several hydrated magnesium ions are observed within the tRNAs. Accession codes: Atomic coordinates and structure factors for the LeuRS Ec ·tRNA·TM84 ternary complex have been deposited in the RCSB Protein Data Bank under accession code 3zgz . How to cite this article: Chopra, S. et al . Plant tumour biocontrol agent employs a tRNA-dependent mechanism to inhibit leucyl-tRNA synthetase. Nat. Commun. 4:1417 doi: 10.1038/ncomms2421 (2013).